Ionizing irradiation induces acute haematopoietic syndrome and gastrointestinal syndrome independently in mice The role of bone marrow (BM) and BM-derived cells in radiation-induced acute gastrointestinal (GI) syndrome is controversial. Here we use bone marrow transplantation (BMT), total body irradiation (TBI) and abdominal irradiation (ABI) models to demonstrate a very limited, if any, role of BM-derived cells in acute GI injury and recovery. Compared with WT BM recipients, mice receiving BM from radiation-resistant PUMA KO mice show no protection from crypt and villus injury or recovery after 15 or 12 Gy TBI, but have a significant survival benefit at 12 Gy TBI. PUMA KO BM significantly protects donor-derived pan-intestinal haematopoietic (CD45+) and endothelial (CD105+) cells after IR. We further show that PUMA KO BM fails to enhance animal survival or crypt regeneration in radiosensitive p21 KO-recipient mice. These findings clearly separate the effects of radiation on the intestinal epithelium from those on the BM and endothelial cells in dose-dependent acute radiation toxicity. Acute radiation exposure can cause lethal injuries to the haematopoietic (HP) and gastrointestinal (GI) systems depending on the dose [1] . The small intestine is one of the most rapidly renewing tissues in mammals, with the intestinal epithelium turning over every 3–5 days in mice in a process fueled by the intestinal stem cells (ISCs) [1] , [2] . Maintenance and self renewal of ISCs are governed by both intrinsic as well as niche signalling during homoeostasis or regeneration on injury [3] , [4] . In the setting of the GI syndrome, ISCs are killed through apoptotic and non-apoptotic mechanisms that are regulated by the p53 pathway [5] , [6] , [7] , [8] . In mice, bone marrow transplantation (BMT) post radiation rescues the HP syndrome but not GI syndrome caused by radiation doses at or above 14 Gy, or LD 50/10 or LD 50/7 doses [9] , [10] . Radiation depletes or inhibits non-epithelial cells such as the BM [9] , endothelial cells [11] , [12] and intestinal subepithelial myofibrobalsts [13] . Various growth factors including fibroblast growth factor-2, insulin-like growth factor-1, keratinocyte growth factor and R-spondin1 improve crypt survival and regeneration, and can be systemically induced by BM-derived cell transplantation [11] , [14] , [15] , [16] , [17] . In addition, BM-derived cells might contribute to tissue regeneration after injury by direct incorporation. In BM transplanted recipients, BM-derived cells are found incorporated into cardiac and skeletal muscle, vascular endothelium and neuronal tissues [18] , [19] , [20] . BM-derived cells were found to be incorporated at very low frequency (~1%), and at slightly increased rates during periods of high proliferation following injury [21] , while other studies suggest such cells rarely transdifferentiate into intestinal epithelium [22] , [23] . Therefore, it remains unclear whether injury to the BM or BM-derived cells contributes to the GI syndrome and associated acute epithelial injury and regeneration [24] . PUMA is a BH3-only proapoptotic Bcl-2 family protein, and kept at very low levels in resting cells. In response to stress, PUMA is rapidly induced through both p53-dependent and -independent manners to promote apoptosis [25] , [26] . Biochemically, PUMA antagonizes all five known antiapoptotic Bcl-2 members through high-affinity protein–protein interactions to initiate apoptosis via the mitochondria [26] . We and others have previously shown that p53-dependent PUMA induction mediates radiation-induced GI and HP injury and syndrome [5] , [27] , [28] . PUMA knockout (KO) mice are highly resistant to radiation-induced HP injury, and wild-type (WT) mice transplanted with PUMA KO BM can survive two doses of 9 Gy total body irradiation (TBI) beyond 18 months without developing leukaemia [27] , [29] . We therefore took advantage of highly radioresistant PUMA KO BM to address the potential BM contribution to the GI syndrome. Using BMT models, we track the survival and responses of BM-derived cells and epithelial cells after ionizing radiation in the intestinal tract of mice. We use TBI and abdominal irradiation (ABI) models, as well as BM donors and recipients with varying sensitivities. Our data demonstrate a very limited, if any, role of BM-derived cells in the GI syndrome and associated acute GI injury and regeneration, and strongly support epithelial and stem cell injury as the primary cause. PUMA KO BM transplant fails to protect against GI syndrome PUMA deficiency protected mice against the GI syndrome following 15 and 18 Gy TBI [5] , [6] , and against the HP syndrome following 6–10 Gy TBI [27] , [28] , [29] . To specifically address the BM contributions to GI injury, we ablated the BM of C57BL/6 WT-recipient mice with 10 Gy TBI followed by transplantation with either WT or apoptosis-resistant ( PUMA KO) whole or CD45 + BM. Following engraftment at 8 weeks, mice were irradiated with 15 Gy TBI and analysed for survival. We found that PUMA KO whole or CD45 + BM did not prolong the survival of recipient mice ( Fig. 1a,b ). Green fluorescence protein (GFP)-positive or -negative donor marrow had no influence on the survival of transplanted mice following radiation ( Supplementary Fig. 1 ). These results strongly suggest that GI, not BM, damage is the primary cause of lethality. 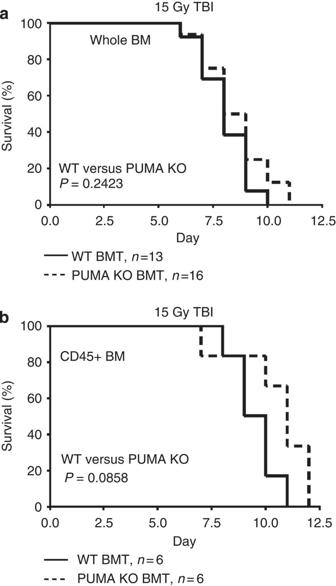Figure 1: Apoptosis-resistant BM does not prolong survival of mice after 15 Gy TBI. Kaplan–Meier survival curves of (a) WT andPUMAKO BMT recipients and (b) WT andPUMAKO CD45+BMT recipients exposed to 15 Gy TBI.Pvalues were calculated by log-rank test. Figure 1: Apoptosis-resistant BM does not prolong survival of mice after 15 Gy TBI. Kaplan–Meier survival curves of ( a ) WT and PUMA KO BMT recipients and ( b ) WT and PUMA KO CD45 + BMT recipients exposed to 15 Gy TBI. P values were calculated by log-rank test. Full size image PUMA KO does not affect BM contribution in the intestine To specifically examine BM influence on the intestinal tract, we examined BM (GFP + ) contribution to several major cell types in the crypts and villi ( Fig. 2a ). Double staining of the epithelial marker cytokeratin and GFP indicated little epithelial contribution (less than 4%; Fig. 2b ; Table 1 ). BM contribution to the CD45 + (pan-HP; 76–95%) and CD105 + (endothelial; 74–89%) populations was dominant and slightly higher with whole BM than CD45 + BMT ( Fig. 2c,d and Supplementary Fig. 2a,b ; Table 1 ). Only a minor BM contribution (less than 10%) to α-smooth muscle actin (α-SMA) + cells (myofibroblasts) was observed ( Fig. 2e and Supplementary Fig. 2c ; Table 1 ). In the crypts, no CD45+ BM contribution was found in myofibroblasts (α-SMA + ) or epithelial cells (cytokeratin + ). The engraftment efficiencies of these four cell types were not affected by the PUMA genotype ( Table 1 ). These data demonstrate that the BM only contributes to a few non-epithelial cells in the small intestine. 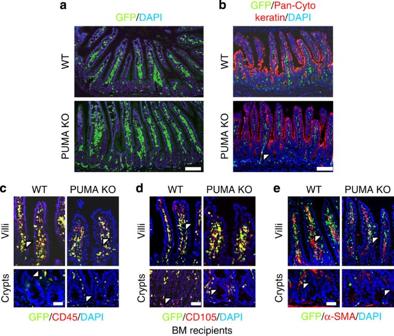Figure 2: Contribution of transplanted BM to the small intestine. WT andPUMAKO BMT (GFP+) recipients. (a) IF demonstrating GFP+BM engraftment in the small intestine. Scale bar, 100 μm. (b) GFP/cytokeratin-double IF identifying donor-derived intestinal epithelium. Scale bar, 100 μm. (c) GFP/CD45-double IF identifying donor-derived CD45+cells in the crypt and villus regions. Scale bar, 50 μm. (d) GFP/CD105-double IF identifying donor-derived CD105+cells in the crypt and villus regions. Scale bar, 50 μm. (e) GFP/α-SMA-double IF identifying donor-derived α-SMA+cells (fibroblasts) in the crypt and villus regions. Arrowheads indicate GFP/lineage double-positive cells. Scale bar, 50 μm. Images are representative forn=3 mice per group. Figure 2: Contribution of transplanted BM to the small intestine. WT and PUMA KO BMT (GFP + ) recipients. ( a ) IF demonstrating GFP + BM engraftment in the small intestine. Scale bar, 100 μm. ( b ) GFP/cytokeratin-double IF identifying donor-derived intestinal epithelium. Scale bar, 100 μm. ( c ) GFP/CD45-double IF identifying donor-derived CD45 + cells in the crypt and villus regions. Scale bar, 50 μm. ( d ) GFP/CD105-double IF identifying donor-derived CD105 + cells in the crypt and villus regions. Scale bar, 50 μm. ( e ) GFP/α-SMA-double IF identifying donor-derived α-SMA + cells (fibroblasts) in the crypt and villus regions. Arrowheads indicate GFP/lineage double-positive cells. Scale bar, 50 μm. Images are representative for n =3 mice per group. Full size image Table 1 Contribution of transplanted BM in the small intestine. Full size table PUMA KO BM does not suppress epithelial damage We then examined intestinal injury and regeneration after 15 Gy TBI in WT and PUMA KO BMT recipients. No difference was observed between WT and PUMA KO BMT mice in crypt apoptosis ( Fig. 3a,b ), proliferation ( Fig. 3c,d ) or regeneration ( Fig. 3e,f ), or between WT or PUMA KO CD45+ BMT mice ( Supplementary Fig. 3a–e ). CD166, a marker for the ISC niche, which stains both Paneth cells and ISCs [30] , decreased similarly in WT and PUMA KO BMT mice ( Fig. 3g,h ). Extremely rare GPF+ epithelial events (GFP+/cytokeratin+, less than 0.1%) were observed in the regenerated crypts in WT and PUMA KO BMT mice ( Supplementary Fig. 3f ). 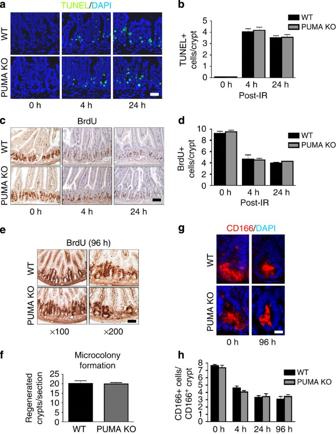Figure 3: Apoptosis-resistant BM does not alter intestinal crypt response to 15 Gy TBI. WT andPUMAKO BMT recipients were exposed to 15 Gy TBI. (a) TUNEL IF in BMT mice at the indicated times. ( × 200 magnification). Scale bar, 50 μm. (b) Quantification of TUNEL-positive cells in intestinal crypts of mice treated as ina. (c) BrdU incorporation in the transplanted mice at the indicated times. ( × 100 magnification); scale bar, 100 μm. (d) Quantification of BrdU-positive cells in intestinal crypts of mice treated as ina. (e) BrdU staining labelled regenerated crypts in transplanted mice. Scale bar, 50 μm. (f) Quantification of regenerated crypts frome. (g) CD166 IF in intestinal crypts of transplanted mice. ( × 400 magnification). Scale bar, 25 μm. (h) Quantification of CD166+cells in CD166+crypts at the indicated times. Values inb,d,fandhrepresent means+s.d. forn=3 mice per group. Figure 3: Apoptosis-resistant BM does not alter intestinal crypt response to 15 Gy TBI. WT and PUMA KO BMT recipients were exposed to 15 Gy TBI. ( a ) TUNEL IF in BMT mice at the indicated times. ( × 200 magnification). Scale bar, 50 μm. ( b ) Quantification of TUNEL-positive cells in intestinal crypts of mice treated as in a . ( c ) BrdU incorporation in the transplanted mice at the indicated times. ( × 100 magnification); scale bar, 100 μm. ( d ) Quantification of BrdU-positive cells in intestinal crypts of mice treated as in a . ( e ) BrdU staining labelled regenerated crypts in transplanted mice. Scale bar, 50 μm. ( f ) Quantification of regenerated crypts from e . ( g ) CD166 IF in intestinal crypts of transplanted mice. ( × 400 magnification). Scale bar, 25 μm. ( h ) Quantification of CD166 + cells in CD166 + crypts at the indicated times. Values in b , d , f and h represent means+s.d. for n =3 mice per group. Full size image Villus height and crypt numbers are sensitive measures of stem cell or progenitor output and crypt survival after radiation, respectively [1] . The extent of villus shortening and crypt loss was identical in BMT groups within 4 days after 15 Gy TBI ( Supplementary Fig. 4a,c ). In contrast, PUMA KO mice showed increased villus height and crypt numbers compared with WT mice, indicating improved epithelial and stem cell survival and recovery ( Supplementary Fig. 4b,d ). BMT WT mice started with significantly shorter villi (385 versus 525 μM) but slightly fewer crypts (118 versus 128), compared with non-BMT mice ( Supplementary Fig. 4 ). These data indicate that PUMA KO-mediated intestinal protection is independent of the BM or BM-derived niche cells. PUMA KO protects BM-derived non-epithelial cells In contrast to the findings in the epithelium, PUMA KO BM significantly suppressed irradiation-induced apoptosis in the villi ( Fig. 4a,b ). Greater numbers of CD45 + pan-HP cells or CD105 + endothelial cells were found in the villi in PUMA KO BMT recipients after radiation ( Fig. 4c–f ), which were associated with reduced apoptosis ( Supplementary Fig. 5 ). The numbers of myofibroblasts (α-SMA + ) did not decrease or differ between these groups around the crypts or villi after irradiation ( Fig. 4g–i ), consistent with a minor BM contribution ( Table 1 and Fig. 2 ). Therefore, PUMA KO confers radioresistance and apoptosis resistance to BM-derived cells in the small intestine. Together with the lack of survival or epithelial benefit in PUMA KO BMT mice ( Figs 1 and 3 ), our data strongly suggest epithelial cell damage is the primary driver of GI syndrome and associated injury [6] , [7] . 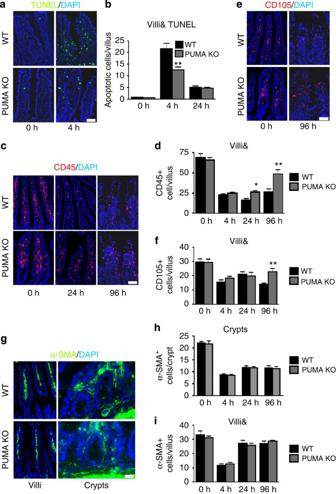Figure 4: Apoptosis-resistant BM protects stroma following 15 Gy TBI. BMT mice were treated as inFig. 3. (a) TUNEL IF in intestinal villi of BMT mice ( × 200 magnification). Scale bar, 25 μm. (b) Quantification of TUNEL+cells in intestinal villi (&, corrected for villus height) at the indicated times following 15 Gy TBI. (c) CD45 IF in intestinal villi of BMT mice at the indicated times ( × 200 magnification). Scale bar, 50 μm. (d) Quantification of CD45+cells in intestinal villi at the indicated times following 15 Gy TBI. (e) CD105 IF in intestinal villi of BMT mice ( × 200 magnification). Scale bar, 50 μm. (f) Quantification of CD105+cells in intestinal villi at the indicated times following 15 Gy TBI. (g) α-SMA IF in intestinal villi of BMT mice ( × 200 magnification). Scale bar, 25 μm. (h) Quantification of α-SMA+cells in intestinal crypts at the indicated times following 15 Gy TBI. (i) Quantification of α-SMA+cells in intestinal villi at the indicated times following 15 Gy TBI. &, quantification inb,d,fandiwas corrected for villus height as shown inSupplementary Fig. 4, and values represent means+s.d. forn=3 mice per group. *P<0.05, **P<0.01 (Student’st-test, two-tailed). Figure 4: Apoptosis-resistant BM protects stroma following 15 Gy TBI. BMT mice were treated as in Fig. 3 . ( a ) TUNEL IF in intestinal villi of BMT mice ( × 200 magnification). Scale bar, 25 μm. ( b ) Quantification of TUNEL + cells in intestinal villi (&, corrected for villus height) at the indicated times following 15 Gy TBI. ( c ) CD45 IF in intestinal villi of BMT mice at the indicated times ( × 200 magnification). Scale bar, 50 μm. ( d ) Quantification of CD45 + cells in intestinal villi at the indicated times following 15 Gy TBI. ( e ) CD105 IF in intestinal villi of BMT mice ( × 200 magnification). Scale bar, 50 μm. ( f ) Quantification of CD105 + cells in intestinal villi at the indicated times following 15 Gy TBI. ( g ) α-SMA IF in intestinal villi of BMT mice ( × 200 magnification). Scale bar, 25 μm. ( h ) Quantification of α-SMA + cells in intestinal crypts at the indicated times following 15 Gy TBI. ( i ) Quantification of α-SMA + cells in intestinal villi at the indicated times following 15 Gy TBI. &, quantification in b , d , f and i was corrected for villus height as shown in Supplementary Fig. 4 , and values represent means+s.d. for n =3 mice per group. * P <0.05, ** P <0.01 (Student’s t -test, two-tailed). Full size image PUMA KO BM protection does not affect GI injury We further separated the BM and GI toxicity after 12 Gy TBI using BMT and non-BMT mice. Despite significant BM protection and survival benefit in PUMA KO BMT or PUMA KO mice, no effect was found on crypt survival in these groups ( Fig. 5 a–f and Supplementary Fig. 6 ). The survival of PUMA KO BMT recipients, who received an additional 10 Gy TBI for BM ablation, was surprisingly close to that of PUMA KO mice ( Fig. 5a,e ). However, crypt apoptosis was significantly suppressed in PUMA KO but not PUMA KO BMT mice, while villus shortening is not affected ( Fig. 5c,d,g,h and Supplementary Fig. 6c,d ). This argues that most crypt apoptosis following 12 Gy TBI carries little functional consequence in the ISC compartment, and perhaps is limited in the progenitor and transient amplifying cells, evident by a minor reduction in crypt numbers (110–103) ( Fig. 5b–d,g,h ). 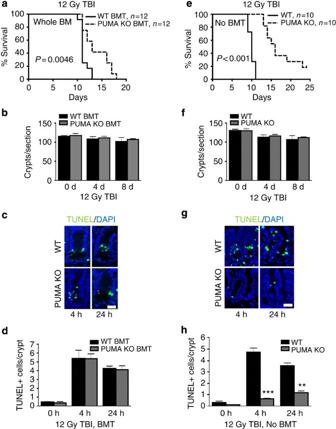Figure 5: Improved animal survival and BM function do not alter GI radiation responses after 12 Gy TBI. (a–d) WTor PUMAKO BMT recipients were analysed at indicated times for animal survival, crypt survival and apoptosis. (a) The Kaplan–Meier survival curve of BMT recipients. (b) Quantification of total crypts per cross-section of BMT mice.n=2 mice per group. (c) Representative images of TUNEL IF in BMT mice ( × 400 magnification). Scale bar, 25 μm. (d) Quantification of TUNEL in intestinal crypts of mice inc.n=3 mice per group. (e–h) WT orPUMAKO mice were exposed to 12 Gy TBI and analysed as ina–d.a,ewere analysed by log-rank test. Values inbandfanddandhrepresent means+s.e.m., and means+s.d., respectively. **P<0.01, ***P<0.001 (Student’st-test, two-tailed). Figure 5: Improved animal survival and BM function do not alter GI radiation responses after 12 Gy TBI. ( a – d ) WT or PUMA KO BMT recipients were analysed at indicated times for animal survival, crypt survival and apoptosis. ( a ) The Kaplan–Meier survival curve of BMT recipients. ( b ) Quantification of total crypts per cross-section of BMT mice. n =2 mice per group. ( c ) Representative images of TUNEL IF in BMT mice ( × 400 magnification). Scale bar, 25 μm. ( d ) Quantification of TUNEL in intestinal crypts of mice in c . n =3 mice per group. ( e – h ) WT or PUMA KO mice were exposed to 12 Gy TBI and analysed as in a – d . a , e were analysed by log-rank test. Values in b and f and d and h represent means+s.e.m., and means+s.d., respectively. ** P <0.01, *** P <0.001 (Student’s t -test, two-tailed). Full size image Using 11 Gy TBI, we found no reduction in crypt numbers, villus height and proliferation index in WT BMT mice at day 8 compared with day 0, indicating complete recovery or limited crypt or ISC loss ( Fig. 6 ). Compared with WT BMT mice, PUMA KO BMT mice also had fully recovered villus height, but a slight increase in crypt numbers (10.9%) and crypt proliferation (21%), probably attributable to the BM protection ( Fig. 6 ). Together, these results demonstrate that crypt injury or regeneration is very limited after TBI at 12 Gy or lower despite crypt apoptosis, and the lethality is almost entirely driven by BM failure. 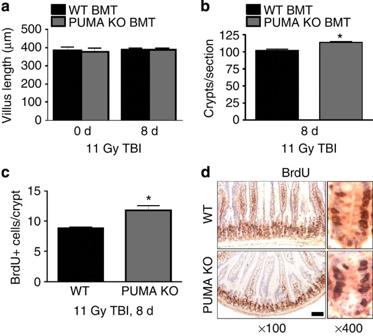Figure 6: Minimal damage or BM influence to the intestinal epithelium after 11 Gy TBI. WT orPUMAKO BMT recipients were analysed at day 8 after 11 Gy TBI. (a) Quantification of intestinal villus height. (b) Quantification of total intestinal crypts per cross-section. (c) Quantification of BrdU-positive cells per intestinal crypt. (d) Representative images of BrdU immunohistochemistry in the small intestine as incat the indicated magnifications. Scale bar, 100 μm. Values ina–crepresent means+s.d. forn=3 mice per group. *P<0.05 (Student’st-test, two-tailed). Figure 6: Minimal damage or BM influence to the intestinal epithelium after 11 Gy TBI. WT or PUMA KO BMT recipients were analysed at day 8 after 11 Gy TBI. ( a ) Quantification of intestinal villus height. ( b ) Quantification of total intestinal crypts per cross-section. ( c ) Quantification of BrdU-positive cells per intestinal crypt. ( d ) Representative images of BrdU immunohistochemistry in the small intestine as in c at the indicated magnifications. Scale bar, 100 μm. Values in a – c represent means+s.d. for n =3 mice per group. * P <0.05 (Student’s t -test, two-tailed). Full size image PUMA KO BM fails to protect p21 KO GI epithelium We then used ABI models and radiosensitive p21 KO mice [6] , [31] as recipients or donors to further determine the role of BM in the GI syndrome. Following 15 Gy ABI, the survival of WT, PUMA KO and p21 KO mice were similar to those after 15 Gy TBI ( Fig. 7a and Supplementary Fig. 7a ) [6] , supporting intestinal damage as the major cause of lethality [5] , [6] . We then generated p21 KO mice with either p21 KO or PUMA KO BM to maximize differences in BM radiosensitivity, and observed no difference in animal survival, and only limited GI toxicity (20% lethality by day 20 and beyond) after 13.5 ABI ( Fig. 7b ). The increased GI sensitivity of the p21 KO mice over WT mice is associated with early and increased crypt regeneration and DNA repair failure [6] . The early and increased crypt regeneration was preserved in the p21 KO BMT mice after 15 Gy TBI, compared with the WT BMT recipients, irrespective of the BM donor ( Fig. 7c,d and Supplementary Fig. 7b,c ). These data clearly indicate that animal survival, and the timing or level of ISC regeneration in the context of the GI syndrome operates independently from the BM. 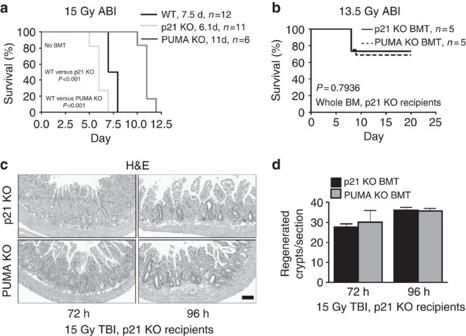Figure 7: Apoptosis-resistant BM does not improve survival or crypt regeneration in radiosensitive hosts. (a) The Kaplan–Meier survival curve of non-transplanted WT,PUMAKO andp21KO mice exposed to 15 Gy ABI. (b)p21KO orPUMAKO BMTp21KO recipients. The Kaplan–Meier survival curve of the BMT mice exposed to 13.5 Gy ABI. (c) H&E staining of intestinal sections fromp21KO BMT mice at the indicated times after exposure to 15 Gy TBI. ( × 100 magnification). Scale bar, 100 μm. (d) Quantification of regenerated crypts in BMT mice treated as inc.aandbwere analysed by log-rank test. Values indrepresent means+s.d. forn=3 mice per group. Figure 7: Apoptosis-resistant BM does not improve survival or crypt regeneration in radiosensitive hosts. ( a ) The Kaplan–Meier survival curve of non-transplanted WT, PUMA KO and p21 KO mice exposed to 15 Gy ABI. ( b ) p21 KO or PUMA KO BMT p21 KO recipients. The Kaplan–Meier survival curve of the BMT mice exposed to 13.5 Gy ABI. ( c ) H&E staining of intestinal sections from p21 KO BMT mice at the indicated times after exposure to 15 Gy TBI. ( × 100 magnification). Scale bar, 100 μm. ( d ) Quantification of regenerated crypts in BMT mice treated as in c . a and b were analysed by log-rank test. Values in d represent means+s.d. for n =3 mice per group. Full size image Acute radiation exposure can lead to the GI syndrome at doses higher than that required for inducing the HP syndrome, and is associated with significant loss of crypts, ISCs and other cell types [1] , [8] , [32] . Adult tissue stem cells are regulated by both cell autonomous and non-cell autonomous signalling, and the BM and BM-derived cells have been suggested to modulate radiation-induced intestinal injury and lethality. Even recent work suggests that blocking endothelial cell apoptosis protects against GI syndrome [33] , [34] , while a clear protection of the crypt cells is not adequately considered. In this study, we presented strong evidence to support that the radiosensitivity of the BM or BM-derived cells does not influence that of the GI epithelium. Our findings together with earlier studies [1] , [5] , [6] , [7] , [35] demonstrate that acute intestinal injury and the GI syndrome are driven by epithelial injury via cell autonomous mechanisms [8] . These findings help better understand the discrete cellular targets and dose responses in acute radiation toxicity, and facilitate the development of countermeasures. PUMA KO mice are the most radioresistant mice to our knowledge, highly protected from BM and GI injury caused by 4–18 Gy TBI [5] , [27] , [28] . The BMT model offers a unique system to separate the effects of PUMA KO in the BM and GI. PUMA KO BM does not affect the reconstitution of the BM-derived intestinal niche including HP (CD45+) or endothelial (CD105+) populations and provides protection to these populations. In contrast, PUMA KO BM did not influence crypt apoptosis, survival, regeneration or villus height, irrespective of BM protection and survival benefit (15, 12 and 11 Gy) in recipients. Moreover, PUMA KO BM fails to alter irradiation-induced lethality, or the extent or kinetics of crypt regeneration in radiosensitive p21 KO recipients at GI relevant doses (13.5 ABI and 15 Gy TBI). It is likely that increased survival of PUMA KO BMT mice, compared with WT BMT mice, will be observed between 12 and 15 Gy, while any impact on the GI epithelial injury or regeneration is highly unlikely and absent at either 12 or 15 Gy. It is also possible, although extremely unlikely, that higher levels of BM protection than what PUMA KO provides are required to protect against radiation-induced acute GI injury. In addition, signalling between the BM, BM-derived cells or factors and the crypt or rare fusion events [22] , [23] are also unlikely to play a significant role in epithelial or ISC injury or regeneration in the context of GI syndrome. Our data shed some light to several long standing and puzzling observations. Crypt apoptosis is not always associated with animal survival or epithelial injury, and is induced by even 1–2 Gy TBI, while the villi can fully recover even after 8 Gy (refs 1 , 5 ) to 11 Gy (this study) in 1–2 weeks. Our data suggest that ISCs, unlike radiosensitive progenitors or transient amplifying cells, are highly resistant to radiation even at 12 Gy TBI. Further, over 50% of PUMA KO BMT recipients survived a total of 28 Gy TBI beyond 18 months without cancer [7] , [29] . These data help explain a dose-dependent sharp drop of survival following TBI at higher doses (above 13.5 or 14 Gy), when the targets are switched to the ISCs, and therefore the limited efficacy of HP cell (CD45 + cells) or BM-derived stromal cell (CD45 − ) transplantation in humans [36] or mice [9] , [37] , [38] . At 12 Gy or lower TBI, the lethality is almost completely driven by the HP syndrome in C57BL/6 mice, cautioning a need to critically evaluate published work on GI injury and protection using such doses. Our data therefore strongly argue against a role of the BM in the GI syndrome, while support that BM injury contributes to delayed radiation enteropathy (11 Gy data) [39] , [40] . Our findings have important implications for the development of radioprotectors and mitigators for the GI syndrome. Many agents including antioxidants, growth factors and Toll-like receptor agonists such as CBLB502 (ref. 41 ) can prolong the survival of mice after TBI, and protect the GI epithelium, BM and among other tissues, yet only a few protect against the GI syndrome (14 Gy or higher) [8] , [32] . Almost all of these agents are more effective when given before radiation, and several of them suppress radiation-induced apoptosis in the crypts and ISCs [16] . Additional mechanisms such as p21-dependent checkpoint and DNA repair are important for intestinal radioprotection in PUMA KO mice [6] and the ‘super p53’ mice [42] . It is also important to balance normal tissue protection with cancer risk. Unlike p53 KO or Bcl-2 transgenic mice, PUMA KO mice or BMT mice do not show elevated risk for leukaemia [27] , [29] . Therefore, simultaneously improving ISC survival and DNA repair, perhaps with small-molecule CDK [43] and PUMA inhibitors [44] , could be efficacious. Mice and treatment The procedures for all animal experiments were approved by the Institutional Animal Care and Use Committee of the University of Pittsburgh. The generation and use of PUMA KO [5] , [45] , p21 KO [6] , [31] , GPF transgenic (WT/GFP+; The Jackson Laboratory, Bar Harbor, ME) and PUMA KO/GFP+ mice [27] have been described. All strains are in or have been back crossed to the C57BL/6 background for more than 10 generations (F10). Mice were generated from heterozygote breeding for PUMA KO genotype, and homozygote breeding for p21 KO. Mice were housed in micro-isolator cages in a room illuminated from 07:00 to 19:00 hours (12:12-h light–dark cycle), with access to water and chow ad libitum . Genotyping of WT, PUMA KO [46] and p21 KO [31] alleles were performed by PCR amplification of genomic DNA purified from tail snips, using the following primers: PUMA KO (1) 5′-TTATAGCCGGTGAGTCAGCA, (2) 5′-TTGACGAGTTCTTCTGAGGG, (3) 5′-CAGGCAGTTGTCAGCTGGG; p21 KO (1) 5′-AAGCCTTGATTCTGATGTGGGC, (2) 5′-TGACGAAGTCAAAGTTCCACCG, (3) 5′-GCTATCAGGACATAGCGTTGGC. TBI was administered at a rate of 76 cGy min −1 in a 137 Cs irradiator (Mark I, JL Shepherd and Associates, San Fernando, CA, USA). ABI was administered in the form of X-ray with a clinical grade linear accelerator (Varian Medical Systems, Palo Alto, CA, USA). For ABI experiments, a 3-cm wide radiation band was used to deliver the required dose at a rate of 600 Monitor Units (146 cGy min −1 ) to anaesthetized animals in groups of 10–15 per run. Following radiation, mice were housed in autoclaved cages and fed only autoclaved food and water to prevent infection. Non-transplanted mice of both genders were irradiated at age 7–9 weeks, while BMT-recipient female mice were irradiated at age 15–17 weeks. BMT and analyses Seven- to 9-week-old female C57BL/6 mice (The Jackson Laboratory) received 10 Gy TBI the day before transplantation. The following morning, ~1 × 10 6 cells (whole marrow or CD45 + cells, as indicated) from 7–9-week-old male C57BL/6 donors were transplanted intravenously via tail vein injection [27] . Donor marrow was harvested from the femurs of WT, PUMA KO or p21 KO mice with or without GFP transgene as indicated. For some experiments, 1 × 10 6 CD45+ BM cells were used in transplantation, which were isolated by flow cytometry following staining with fluorescein isothiocyanate-labelled anti-CD45 (1:100, 553080; BD Biosciences, San Jose, CA) [27] . Following transplantation, mice were allowed 8 weeks for engraftment after which they were irradiated a second time, as indicated, and followed for survival or harvested at multiple time points for tissue analysis. Tissue processing All mice were injected with 100 mg kg −1 5-bromo-2'-deoxyuridine (BrdU; Sigma-Aldrich, St Louis, MO) 2 h before killing. Immediately after the killing, an ~10 cm jejunum was removed and carefully rinsed with ice-cold saline. The tissue was either cut into 6–8 sections (1 cm) and bundled with 3 M micropore tape, or opened longitudinally and tacked to a foam board. Both preparations were fixed overnight in 10% formalin. Tissues processed either as bundles or ‘Swiss rolls’ were then embedded in paraffin and sectioned. Five micrometres thick sections were used for haematoxylin and eosin (H&E) staining and immunodetection of various proteins and markers. Crypt microcolony assay The crypt microcolony assay was used to quantify stem cell survival by counting regenerated crypts in H&E-stained cross-sections 4 days post irradiation [5] , [47] , [48] . Surviving crypts were defined as containing five or more adjacent chromophilic non-Paneth cells, at least one Paneth cell and a lumen. The number of surviving crypts was counted in 6–8 circumferences per mouse, with each ~1 cm apart. BrdU staining was also used to quantify regenerated crypts. The regenerated crypts contained five or more BrdU-positive cells with a lumen. The numbers of regenerated crypts scored by these two methods were similar. The data from BrdU staining was reported as means±s.e.m. ( n =2 mouse per group) or ±s.d. ( n =3 mice per group). Villus height measurements Average villus height was determined by measuring 30–40 villi from different locations of the small intestine, from at least two different animals per group and reported as means±s.e.m. Measurements were made from the top of crypt to the tip of the villus using × 100 H&E images and SPOT 5.1 Advanced software (Diagnostic Instruments Inc., Sterling Heights, MI). Immunohistochemistry and immunofluorescence (IF) Immunodetection of various proteins and markers was performed following deparaffinization and antigen retrieval. Antigen retrieval was performed by boiling sections for 10 min in 0.1 M citrate buffer (pH 6.0) with 1 mM EDTA. TUNEL IF and BrdU immunohistochemistry Terminal deoxynucleotidyl transferase dUTP nick-end labelling (TUNEL) staining was conducted with the ApopTag Fluorescein In Situ Apoptosis Detection Kit (Millipore, Billerica, MA) according to the manufacturer’s instructions. For BrdU staining, sections were treated with proteinase K (20 μg ml −1 ) for 20 min at 37 °C. Staining was carried out following a standard peroxidase protocol with an anti-BrdU antibody (A21301MP, Invitrogen, Carlsbad, CA; 1:100 in 10% goat serum), secondary antibody (goat-anti-mouse-biotin, 1:100; #31802; Pierce, Rockford, IL), and then amplified with the VectaStain ABC kit and developed by 3,3′-Diaminobenzidine (DAB) (Vector Laboratories, Burlingame, CA). GFP IF Non-specific antibody binding was blocked using 20% goat serum at room temperature for 30 min. Sections were incubated overnight at 4 °C in a humidified chamber with 1:50 diluted mouse-anti-GFP (sc-9996; Santa Cruz Biotechnology, Santa Cruz, CA). Sections were then incubated with AlexaFluor 594-conjugated goat-anti-mouse secondary antibodies (1:200; AA11005; Invitrogen) for 1 h at room temperature and counterstained with VectaShield+4',6-diamidino-2-phenylindole (DAPI; Vector Laboratories). CD166 IF Non-specific antibody binding was blocked using 20% rabbit serum at room temperature for 30 min. Sections were incubated overnight at 4 °C in a humidified chamber with goat-anti-mouse CD166 antibodies (1:100; AF1172; R&D Systems, Minneapolis, MN). Sections were then incubated with AlexaFluor-594 rabbit-anti-goat secondary antibodies (1:100; A11080; Invitrogen) for 1 h at room temperature and counterstained with VectaShield plus DAPI. GFP/TUNEL-double IF Sections were prepared and stained as described for GFP, but before counterstaining, sections were washed with PBS and stained for TUNEL with the ApopTag Fluorescein Kit (Millipore) according to the manufacturer’s instructions. Sections were then counterstained as described. GFP/CD45-double IF Sections were prepared as described and stained for GFP (1:100; ab13970; Abcam; Cambridge, MA) and developed with AlexaFluor-488-conjugated rabbit-anti-chicken secondary antibodies (1:200; 303-545-003: The Jackson Laboratories) for 1 h at room temperature. Slides were then washed in PBS and incubated overnight with rat anti-mouse CD45 antibodies (1:50; 553076; BD Biosciences). Sections were then incubated with AlexaFluor-594 goat-anti-rat secondary antibodies (1:100; A11007; Invitrogen) for 1 h at room temperature and counterstained with VectaShield plus DAPI (Vector Laboratories). GFP/CD105-double IF Sections were prepared and stained for GFP as described for GFP/CD45-double IF. Slides were then washed in PBS and incubated overnight with rat anti-mouse CD105 antibodies (1:50; 14-1051-82; eBioscience, San Diego, CA). Sections were then incubated with AlexaFluor-594 goat-anti-rat secondary antibodies (1:100; A11007; Invitrogen) for 1 h at room temperature and counterstained with VectaShield plus DAPI (Vector Laboratories). GFP/α-SMA-double IF Sections were prepared and stained for GFP as described for GFP/CD45-double IF. Slides were then washed in PBS and incubated overnight with mouse anti-smooth muscle actin (α-SMA) (1:100; MAB1522; Millipore). Sections were then incubated with AlexaFluor-594 goat-anti-mouse secondary antibodies (1:200) for 1 h at room temperature and counterstained with VectaShield plus DAPI (Vector Laboratories). GFP/cytokeratin-double IF Sections were prepared and stained for GFP as described for GFP/CD45-double IF. Slides were then washed in PBS and incubated overnight with mouse-anti-pan-cytokeratin (ab961; AE1+AE3; prediluted; Abcam). Sections were then incubated with AlexaFluor 594-conjugated goat-anti-mouse secondary antibodies for 1 h at room temperature and counterstained with VectaShield+DAPI (Vector Laboratories). CD45/TUNEL-double IF Sections were prepared and stained for CD45 as described. Following incubation with AlexaFluor-594 goat-anti-rat secondary antibodies, sections were washed in PBS and stained for TUNEL with the ApoAlert DNA Fragmentation Assay Kit (Clontech, Mountain View, CA) according to the manufacturer’s instructions. Sections were then counterstained as described. CD105/TUNEL-double IF Sections were prepared and stained for CD105 as described. Following incubation with AlexaFluor-594 goat-anti-rat secondary antibodies, sections were washed in PBS and stained for TUNEL with the ApoAlert DNA Fragmentation Assay Kit and counterstained as described. Analyses of BM and peripheral blood cells BM H&E staining Femurs were collected from mice at the indicated times and fixed overnight in 10% formalin. Samples were then decalcified overnight in Cal-Ex (Fisher) and rinsed in cold water for 30 min, before storage in 70% ethanol until embedding. Paraffin-embedded bones were sectioned and stained with H&E. Giemsa/May–Grunwald staining of blood smears At the time of killing, blood was collected from mice by cardiac puncture. Small drops of blood (~10–15 μl) were spread on glass slides and allowed to air dry. For staining, slides were incubated for 5 min in May–Grunwald stain (Sigma), followed by 1.5 min incubation in 50 mM PBS, pH 7.2. Slides were then transferred to Giemsa stain (1:20 in distilled water) for 15 min. Following a brief rinse in distilled water, slides were air dried and imaged. Statistical analysis Statistical analyses were carried out using GraphPad Prism IV software. The survival data were analysed by log-rank test. Data were analysed by unpaired t -test or analysis of variance in which multiple comparisons were performed using the method of least significant difference. P values were calculated by the Student’s t -test and were considered significant if P <0.05. The means±s.e.m. or ±s.d. are displayed in the figures. How to cite this article: Leibowitz, B. J. et al. Ionizing irradiation induces acute haematopoietic syndrome and gastrointestinal syndrome independently in mice. Nat. Commun. 5:3494 doi: 10.1038/ncomms4494 (2014).